Correspondence: Reassessing the contribution of natural gas to US CO2emission reductions since 2007 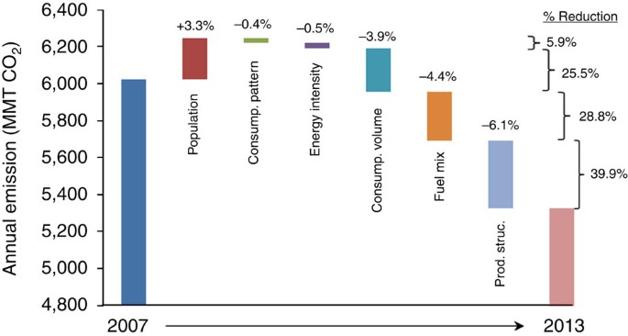Figure 1: Contributions of different factors to the decline of US CO2emissions 2007–2013. Numbers are taken from FDSH’s structural decomposition analysis that spans the whole time period. Changes in the fuel mix are responsible for a 4.4% decrease in energy-related emissions and 28.8% of the emissions decreases that occurred during this period. This amount exceeds that from changes in consumption volume (Consump. volume), but is less than that from changes in production structure (Prod. struct.). 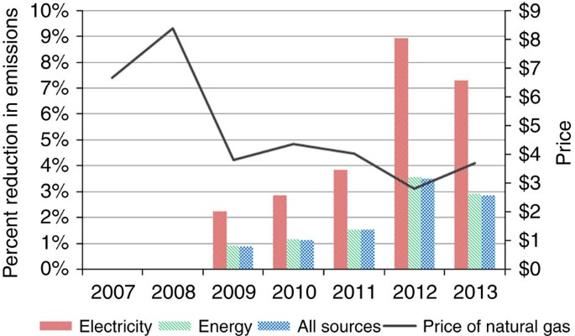Figure 2: Annual percentage reduction of US CO2emissions compared with 2007 levels due to fuel switching of natural gas for coal in electricity generation and annual natural gas prices. Forecasts are based on holding the emission rate from coal and natural gas constant at the 2007 level. Bases for comparison are annual emissions from all fossil-fuel generated electricity, all energy-related emissions and US emissions from all sources. As a share of the overall reduction of emissions from 2007 to 2013 of 10.3%, this method attributes 28.2% to greater use of natural gas in electricity generation. How to cite this article : Kotchen M. J. & Mansur E. T. Correspondence: Reassessing the contribution of natural gas to US CO 2 emission reductions since 2007. Nat. Commun . 7:10648 doi: 10.1038/ncomms10648 (2016).